Using nanoscale and mesoscale anisotropy to engineer the optical response of three-dimensional plasmonic metamaterials The a priori ability to design electromagnetic wave propagation is crucial for the development of novel metamaterials. Incorporating plasmonic building blocks is of particular interest due to their ability to confine visible light. Here we explore the use of anisotropy in nanoscale and mesoscale plasmonic array architectures to produce noble metal-based metamaterials with unusual optical properties. We find that the combination of nanoscale and mesoscale anisotropy leads to rich opportunities for metamaterials throughout the visible and near-infrared. The low volume fraction (<5%) plasmonic metamaterials explored herein exhibit birefringence, a skin depth approaching that of pure metals for selected wavelengths, and directionally confined waves similar to those found in optical fibres. These data provide design principles with which the electromagnetic behaviour of plasmonic metamaterials can be tailored using high aspect ratio nanostructures that are accessible via a variety of synthesis and assembly methods. Metamaterials are artificial materials comprising components smaller than the incident wavelength, which allow for the precise engineering of the spatial and temporal propagation of electromagnetic fields. With the incorporation of nanoscale building blocks, many exciting electromagnetic phenomena are possible at visible wavelengths such as subdiffraction limit lensing [1] , complex mathematics [2] and nanoscale coherent emission sources (lasers) [3] , [4] . Noble metals, the most commonly used plasmonic materials, interact extremely efficiently with visible light and thus are promising candidates for the construction of optically relevant metamaterials [5] , [6] , [7] , [8] , [9] . This strong response arises from the collective oscillation of conduction electrons present in plasmonic nanostructures on excitation [10] . This so-called localized surface plasmon resonance (LSPR) excitation is highly sensitive to the size, shape, composition and local environment of the nanostructure [10] . In addition, shape anisotropy provides a powerful handle for the control of plasmonic electric field enhancement [10] , polarization-dependent response in metamaterial biosensors [11] and for the directed assembly of noble metal nanoparticles [12] , [13] , [14] , [15] , [16] , [17] , [18] , [19] . By arranging anisotropic plasmonic nanoparticles into complex ordered structures, the resulting optical properties can be intelligently designed to vary with polarization, orientation and spectral location, a feat that cannot be reproduced with homogeneous materials. Because of interest in the diverse properties of plasmonic nanostructures, a variety of methods have been developed to assemble them [12] into two-dimensional (2D) and three-dimensional (3D) hierarchical crystalline superlattices, superparticles and superstructures, including DNA-mediated [14] , [20] , [21] , [22] , [23] , drying-forced [24] , [25] , entropically driven [18] , [26] , [27] and electrostatic methods [28] . In addition, recent work on plasmonic nanoparticle clusters suggests that these structures can support magnetic dipole resonances [29] , [30] and Fano lineshapes [31] that are dependent on the cluster size and symmetry. Finally, recent advances in programmable DNA-mediated nanoparticle assembly have produced mesoscale single crystal rhombic dodecahedra [32] , layer-by-layer micron-sized substrates with controlled thickness [33] and methods to lithographically control the size, shape and strain of substrate assembled superlattices [34] . From this, it is clear that assembly control should be thought of on two length scales: nanoscale control over the crystal symmetry, orientation and local arrangement of the nanoparticles; and mesoscale (here taken to mean 100 nm to several microns) control over the overall superlattice structure including crystalline morphology, shape and size. A significant body of work exists concerning nanoscale geometric arrangement and proximity affects on the optical properties of plasmonic nanostructures [10] , [16] , [35] , [36] . For example, extremely anisotropic nanowire arrays have been shown to exhibit ultrafast nonlinearity [37] and birefringence [11] , [38] , where the optical properties differ depending on the incident light polarization. In addition, near-field coupled rod pairs and arrays of rod crosses (in 2D) have been shown to exhibit a negative refractive index in the visible [39] , [40] . However, minimal literature exists exploring the potential optical properties that can arise from the controlling the arrangement of the rich diversity of anisotropic nanoparticles into 3D mesoscale structures. Recently, we have demonstrated that the coupled dipole method (CDM) and Maxwell-Garnett effective medium theory (EMT) provide a powerful combination for predicting properties such as epsilon-near-zero (ENZ) behaviour [41] , [42] (electromagnetic phase attenuation) and an ‘optically metallic’ response (finite skin depth) in DNA-assembled Ag spherical nanoparticle superlattices of arbitrary shape [8] , [9] . The CDM provides a fully retarded electrodynamics solver with which electric fields can be determined for a structure of arbitrary size and shape. EMT is a rapid and general volume fraction-dependent method that can be used to calculate an effective dielectric constant, ε eff. From ε eff , we can gain a physical understanding of how the nanoscale components of resonant media interact with light. However, the mesoscale aspects of these structures have received little attention. In general, these structures can only be considered numerically using the CDM with considerable computational expense and minimal generalizable conclusions. Fortunately, many scattering approximations have been developed to describe the behaviour of objects such as atmospheric water droplets [43] , [44] , microwave antennae [45] and interstellar dust. Anomalous diffraction theory (ADT) [43] is the most relevant approach in this size range (wavelength smaller than the path length of light through an object) and it generally is accurate only when the refractive index is near unity (less than n ~1.3). In ADT, scattering is determined primarily by the phase mismatch between light propagating through the interior of the superlattice crystal and that propagating externally by the object. This approach has been effectively implemented for a variety of materials and shapes [43] , [44] , [45] , [46] , and we will show below that it is useful for describing mesoscale effects for superlattices. In this work, we simulate a proof-of concept that, by combining anisotropic nanoscale components with mesoscale superstructures (that is, sizes in the range 100 nm to a few microns), we can produce a number of unexpected and uniquely tunable optical properties. These include ENZ behaviour, birefringent fast and slow light, and confined and enhanced electromagnetic fields for wavelengths across the visible and near-infrared. Remarkably, at volume fractions of <5%, the skin penetration depths of these materials approach that of pure (100%) noble metals for selected wavelength ranges. Our proposed 3D superstructure surpasses many inorganic crystals that exhibit birefringence or are dichromatic, such as calcite or tourmaline, in that the superstructures’ properties can be engineered to change based on crystal orientation and via polarization control, in addition to being tunable throughout the visible-NIR. Moreover, we verify that the scattering properties of mesoscale plasmonic superlattices are qualitatively described by ADT, with the dominant spectral scattering of plasmonic superlattices dictated by shape effects that ADT describes and with the dielectric function being strongly perturbed even at wavelengths that are hundreds of nanometers from the isolated nanoparticle resonance. Importantly, the nanoparticle building blocks required for these structures can be solution synthesized and in some cases assembled using bottom-up assembly techniques; so our predictions are directly amenable to future experimental studies. Designing optical properties with anisotropy High aspect ratio nanoparticles (HAR-NPs) are of great interest in plasmonics due to the highly tunable and polarization-dependent nature of their LSPR; Fig. 1a depicts a variety of solution synthesized noble metal HAR-NPs including nanorods [47] , [48] , cylindrical disks [49] and triangular nanoprisms [50] , [51] . Because of this interest, a variety of methods have been used to assemble HAR-NPs into arrays [12] , [14] , [15] , [17] , [19] . Importantly, all of these methods orient the NPs in at least one dimension, allowing for a polarization-dependent optical response. Here, we use ellipsoids (more rigorously, spheroids) as a heuristic to describe the resonant properties of superstructures comprising HAR-NPs. 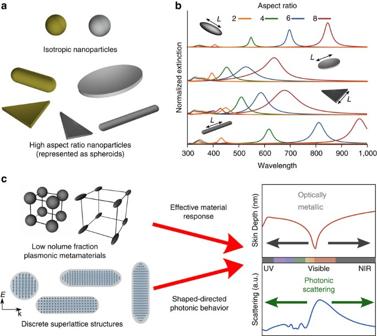Figure 1: Introducing 3D anisotropic nanoparticle superlattices. (a) Examples of isotropic (top) and anisotropic (bottom) noble metal nanoparticles. (b) Spectra of high aspect ratio nanoparticles: ellipsoid (top), cylindrical disk, triangular nanoprism, nanorod (bottom). (c) Scheme depicting the spectral versatility that the combination of nanoscale (top left) and mesoscale (bottom left) architecture provides. Control over nanoscale components provides a handle for controlling the skin depth and collective material resonance (top right), while mesoscale superlattice structure controls photonic resonances and confined optical modes (bottom right). Figure 1: Introducing 3D anisotropic nanoparticle superlattices. ( a ) Examples of isotropic (top) and anisotropic (bottom) noble metal nanoparticles. ( b ) Spectra of high aspect ratio nanoparticles: ellipsoid (top), cylindrical disk, triangular nanoprism, nanorod (bottom). ( c ) Scheme depicting the spectral versatility that the combination of nanoscale (top left) and mesoscale (bottom left) architecture provides. Control over nanoscale components provides a handle for controlling the skin depth and collective material resonance (top right), while mesoscale superlattice structure controls photonic resonances and confined optical modes (bottom right). Full size image Using ellipsoids provides two key advantages: the resonance condition is analytic and can be simulated rapidly, and ellipsoids provide a realistic representation of the longitudinal and transverse resonances of a HAR-NP in the far-field, that is, excluding near-field interactions. Figure 1b depicts spectra of HAR-NPs with fixed short axis lengths (10 nm) and varying long axis lengths (20–80 nm) including ellipsoids (top), cylindrical disks, triangular nanoprisms and nanorods (bottom). Note that, although the exact size-to-resonant wavelength correlation varies, the longitudinal LSPR (solid lines) for all shapes red-shifts with increasing aspect ratio and the transverse LSPR (dashed lines) blue-shifts and weakens in intensity in the UV, near-visible region. Recent experimental LSPR findings suggest that the key determinant of the LSPR spectral location is the length over which the electron oscillations take place, rather than the shape alone [52] . Thus, though the superstructures simulated in this manuscript are comprised solely of ellipsoids, the conclusions and design principles described for creating complex 3D metamaterial superstructures are applicable to the assembly of any plasmonic nanoparticle with a significant aspect ratio. Our studies will focus on controlling optical properties with both mesoscale and nanoscale effects as depicted in Fig. 1c . In the first section, we are concerned with nanoscale anisotropy for cubic lattices, where the nanoparticle structure controls the effective material response. Then we shift to mesoscale anisotropy effects for spherical nanoparticles, where the scattering signature of the superlattice controls optical behaviour. Finally, we incorporate mesoscale anisotropy with anisotropic nanoparticles. To study the optical properties of these mesoscale anisotropic crystals that are composed of anisotropic nanoparticles, we use modifications to the CDM and EMT as detailed in the Methods section. Supplementary Figs 1–4 consider error for both EMT and CDM compared with generalized multiparticle Mie theory (an analytic method) as a function of both superlattice size and Ag volume fraction, the simulated structures are listed in Supplementary Table 1 ; an extended discussion regarding the relative error of these methods can be found in Supplementary Notes 1 and 2 . Anisotropy Effects at the Nanoscale We first focus on the effect of nanoparticle anisotropy by considering cubic lattices composed of HAR-NPs, such as that shown in Fig. 2a . If we recall that ellipsoids oriented longitudinal to the incident field will exhibit a strong LSPR in the visible that red-shifts with increasing aspect ratio, and that transverse oriented ellipsoids will exhibit a weaker LSPR in the UV, then three separate scenarios can occur depending on the orientation of the cube. First, consider Fig. 2b (Orientation 1, left panel), where the ellipsoids are transverse for a 360° azimuthal rotation. In this case, the material response will be polarization independent because the ellipsoids are always transverse to incident light. However, in Orientations 2 and 3 ( Fig. 2b , middle and right panels), the response will be birefringent (polarization-dependent) due to the different ellipsoid orientations on rotation. 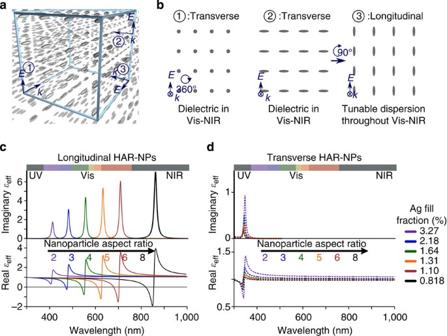Figure 2: A 3D mesoscale superlattice exhibiting both dichromatic and birefringent metamaterial behaviour. (a) A 3D simple cubic arrangement of ellipsoids. (b) The corresponding face projections depicting the possible directions of polarization and propagation. (c) Tunability of the imaginary (top) and real (bottom) effective dielectric function for longitudinally-oriented ellipsoidal media. (d) Tunability of the imaginary (top) and real (bottom) effective dielectric function for transverse-oriented ellipsoidal media. The grey lines depict the zero point. On all plots, the volume fractions correspond to a simple cubic unit cell of ellipsoids of varying aspect ratio with a fixed short axis (10 nm) separated by one long axis length. Figure 2: A 3D mesoscale superlattice exhibiting both dichromatic and birefringent metamaterial behaviour. ( a ) A 3D simple cubic arrangement of ellipsoids. ( b ) The corresponding face projections depicting the possible directions of polarization and propagation. ( c ) Tunability of the imaginary (top) and real (bottom) effective dielectric function for longitudinally-oriented ellipsoidal media. ( d ) Tunability of the imaginary (top) and real (bottom) effective dielectric function for transverse-oriented ellipsoidal media. The grey lines depict the zero point. On all plots, the volume fractions correspond to a simple cubic unit cell of ellipsoids of varying aspect ratio with a fixed short axis (10 nm) separated by one long axis length. Full size image Effective material parameters are useful for predicting and understanding complex optical phenomena for resonant media. Recently, using EMT and the CDM, we predicted that nanoparticle superlattices with ~25% volume fraction of 20 nm diameter Ag nanospheres exhibit both ENZ behaviour and an ‘optically metallic’ skin-depth response at wavelengths close to 400 nm (refs 8 , 9 ) By incorporating ellipsoids, this behaviour can be expanded throughout the visible, taking advantage of the precise tunability of the LSPR in HAR-NPs. The volume fractions stated in Fig. 2 correspond to ellipsoids separated by one major axis length in a simple cubic arrangement. The ellipsoid sizes range from 10 nm short axis × 20 nm long axis, purple trace, to 10 nm short axis × 80 nm long axis, black trace. Supplementary Figure 1 demonstrates that EMT is accurate for these spacings. A full description of our EMT approach can be found in the Methods section, Supplementary Information , and the following references [8] , [53] . Figure 2c,d depicts the imaginary and real parts of the effective dielectric function ε eff , respectively, for an ellipsoidal superlattice media in vacuum. The longitudinal ( Fig. 2c ) and transverse ( Fig. 2d ) effective dielectric functions are plotted separately for convenience. ε eff describes the ability of a material to concentrate electric flux, that is, how much charge it can support. The imaginary part (top plots), Im{ ε eff }, relates to absorption by the structure. The real part (bottom plots), Re{ ε eff }, roughly corresponds to energy stored in the medium. It is from Re{ ε eff } that collective metamaterial properties, such as ENZ and ‘optically metallic’ response, can be understood. Here, we will focus mainly on Re{ ε eff ,}, which determines whether the optical response will be as a dielectric (Re{ ε eff }>0) or as a reflective material (Re{ ε eff }<0); this is also where ENZ (Re{ ε eff }=0) behaviour can be identified. In Fig. 2c , it is seen that for volume fractions of 5% and below, a medium containing longitudinally oriented ellipsoids of aspect ratios of 3–8 exhibits ENZ and Re{ ε eff }<0. In addition, Supplementary Fig. 5 shows the effective response of 2 AR ellipsoids, which have the weakest resonance, in increasing background refractive indices. With increasing background index, the negative well in Re{ ε eff } deepens due to the higher polarizability of Ag nanostructures in higher index media [5] . This suggests that, with the proper tuning of aspect ratio with background index, Re{ ε eff }<0 is attainable throughout the visible-near infrared with a diversity of nanoparticles. The Re{ ε eff }<0 response is achieved at lower volume fractions for ellipsoids than spheres because the ellipsoids are significantly more polarizable than nanospheres at their resonant wavelengths [54] . Also, the polarizability of ellipsoids in the transverse orientation is significantly less than longitudinally oriented ellipsoids, hence Re{ ε eff } ( Fig. 2d , transverse) is minimally dispersive, even on resonance. Because of these orientation-dependent variations in polarizability, we can consider a 3D mesoscale superlattice comprising HAR-NPs as both dichromatic (multi-responsive based on orientation) and birefringent. For Orientation 1 in Fig. 2b , the superlattice will be effectively transparent (neglecting the minor plasmon losses for low volume fraction) and dielectric. In Orientation 2 the superlattice is also a transparent dielectric, but rotation of the polarization to Orientation 3 leads to a tunable ε eff where Re{ ε eff }<0 for tens for nanometers around a selected wavelength range. Note that in a 2D system of ellipsoids (on a substrate, for example) only the birefringent properties would be accessible; the material requires thickness in 3D to exhibit orientation and polarization-dependent properties. A simple way to illustrate how the orientation and polarization dependencies manifest in 3D is via the skin depth, δ SD. The skin depth is a measure of light penetration into a material and can be approximated as where λ is the wavelength and κ is the imaginary part of the refractive index ( m=n+iκ ), a full description can be found in Supplementary Note 3 . The refractive index of the material can be determined from ε eff , obtained from EMT, using the expression, where m is the complex refractive index, ε is the permittivity ( ε eff ) and μ is the permeability ( μ= 1). The real and imaginary components of the refractive index are seen in Supplementary Fig. 6 . Typical skin penetration depths for bulk noble metals (Ag, Au) are <25 nm throughout the vis-NIR. It is seen in Fig. 3a that, for the longitudinal-oriented ellipsoid media, δ SD approaches 10 2 nm when the ellipsoids are on resonance, that is, where the absorption, Im{ ε eff }, is greatest. The 10 2 nm value is ~4 orders of magnitude smaller than when the ellipsoids are off-resonance, where δ SD is ~10 6 nm. Thus, for a mesoscale object on the order of tens of microns in size, the superlattice will be effectively transparent off-resonance but optically thick on-resonance. When δ SD is lowest, these media approach the optical penetration depth of pure Ag metal, even though the volume fraction is very low (<1% for the 8 aspect ratio ellipsoids), and thus over 99% air. For transverse-oriented ellipsoids, Fig. 3b , δ SD is very large (~10 5 –10 7 nm) throughout the vis-NIR, and thus the material can be considered transparent. Only at 360 nm in the UV can the transverse LSPR be excited in which case δ SD is ~10 2 –10 3 nm. A several order of magnitude change in δ SD is also observed in superlattices comprising Au ellipsoids ( Supplementary Fig. 7 ), though the effect is somewhat diminished due to the poorer quality factor of plasmon resonance in Au and some portion of the visible spectral region below 520 nm is distorted due to interband transitions [5] . 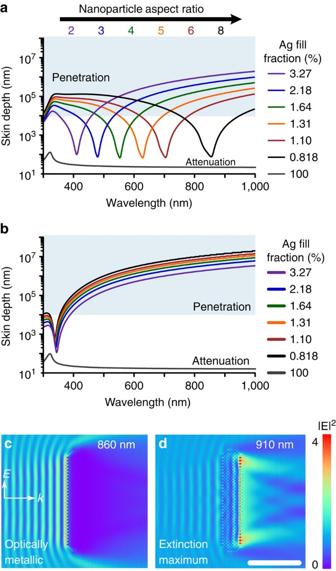Figure 3: Tunability of skin depth in low volume fraction ellipsoidal media. The skin depth for longitudinally oriented, (a) and transverse-oriented (b), ellipsoidal media of varying volume fraction. On both plots, the grey line shows the skin depth for pure Ag metal. The skin depth (left axis) is plotted on a logarithmic scale. Penetration and attenuation of an incident field are demarcated for a micron-scale material. (c) Simulated electric field plot at 860 nm for eight AR ellipsoids in a longitudinal mesoscale superlattice (5,912 nm long by 924 nm wide). (d) Simulated electric field plot at 910 nm for eight AR ellipsoids in a longitudinal mesoscale superlattice. On all plots, the volume fractions correspond to a simple cubic unit cell of ellipsoids of varying aspect ratio with a fixed short axis (10 nm) separated by one long axis length. Scale bar, 2 μm. Figure 3: Tunability of skin depth in low volume fraction ellipsoidal media. The skin depth for longitudinally oriented, ( a ) and transverse-oriented ( b ), ellipsoidal media of varying volume fraction. On both plots, the grey line shows the skin depth for pure Ag metal. The skin depth (left axis) is plotted on a logarithmic scale. Penetration and attenuation of an incident field are demarcated for a micron-scale material. ( c ) Simulated electric field plot at 860 nm for eight AR ellipsoids in a longitudinal mesoscale superlattice (5,912 nm long by 924 nm wide). ( d ) Simulated electric field plot at 910 nm for eight AR ellipsoids in a longitudinal mesoscale superlattice. On all plots, the volume fractions correspond to a simple cubic unit cell of ellipsoids of varying aspect ratio with a fixed short axis (10 nm) separated by one long axis length. Scale bar, 2 μm. Full size image In Fig. 3c,d CDM simulations of the electric field response are shown for rod-like superlattices (5,912 nm long by 924 nm wide) that are longitudinal to the incident polarization. Note that both the nanoparticles and the rod are longitudinal to the incident polarization, and we consider two wavelengths, one where EMT predicts negative dielectric behaviour (at 860 nm in Fig. 3c ) and one corresponding to the extinction maximum for this structure (at 910 nm in Fig. 3d ). In the region where Re{ ε eff }<0, significant attenuation of the incident field is seen with minimal fields in the interior of the superlattice. In addition, significant reflection is also seen at the illuminated face [8] , [42] . In contrast, at the extinction maximum, one sees considerable transmission and far-field focusing of the incident field. This agrees with our previous work on pseudo-randomly shaped superlattices where Re{ ε eff }<0 had both optically metallic regions and an extinction maximum where focusing was primarily seen. It is important to realize here that, although the maximum in Im{ε eff } typically corresponds to the extinction maximum, this is only true within the quasistatic (small particle) limit. Because the structures investigated herein have micron-scale dimensions, the superlattice is no longer quasistatic and it experiences different phases from the incident field at different locations in the superlattice. Because of the mesoscale dimensions of the superlattice, the extinction, Im{ ε eff }, and skin depth minima can vary in behaviour from quasistatic predictions. Thus, it is important to investigate the extinction and scattering behaviour of the superstructures explicitly to fully understand the optical characteristics of a metal nanoparticle superlattice. Anisotropy Effects at the Mesoscale To date, minimal literature exists on the interaction between plasmonic inclusions and mesoscale photonic effects in 3D superlattices. Control of the mesoscale shape alters the scattering signature of the structure, creating effects such as photonic modes and focusing effects akin to those in optical fibres, lenses and photonic crystals. Here we consider the optical response of a mesoscale rod-like superlattice oriented transverse to the incident polarization (SL Trans -Spheres), depicted in Fig. 4a , inset) that is composed of 20 nm diameter Ag nanospheres on a body-centred cubic lattice with a volume fraction ranging from 20.2% Ag (10 nm surface-to-surface gap) to 1.0% Ag (60 nm surface-to-surface gap). These volume fractions were chosen to correlate with recent experimental and theoretical work focusing on the synthesis and characterization of analogous Ag nanoparticle superlattices that were identified as promising plasmonic metamaterial candidates [8] , [9] . The rod-like superlattice size was fixed at a constant 2,000 nm long by 400 nm wide; later other sizes and aspect ratios will be considered. Supplementary Figs 1 – 4 demonstrate the relative accuracy of EMT, the CDM and generalized multiparticle Mie theory (GMM, an analytic solution) for superlattices of varying size and lattice spacing, showing both that EMT is accurate up to volume fractions of ~25% and that superstructure size does not affect the accuracy of either EMT or the CDM. 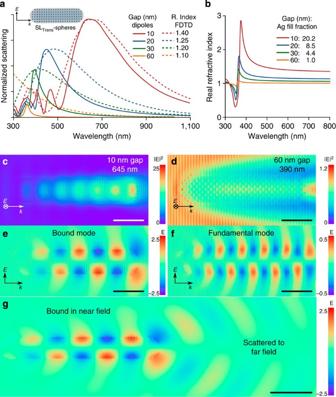Figure 4: Confined electromagnetic radiation due to anomalous diffraction in anisotropic mesoscale superlattices. (a) Simulated 2,000 × 400 nm rod-like superlattice containing dipoles (solid) or a fixed real refractive index value (dashed). Inset depicts the orientation of the superlattices relative to the incident light. (b) Effect of changing interparticle gap (volume fraction) on real refractive index of dielectric media (n=1) with 20 nm Ag spheres. (c) Electric field-squared plot of rod-like superlattice with 10 nm surface-to-surface interparticle gap at the extinction maximum (wavelength=645 nm). (d) Electric field-squared plot of rod-like superlattice with 60 nm surface-to-surface interparticle gap at the extinction maximum (wavelength=390 nm). (e) Absolute electric field plots for 10 nm gap (e) and 60 nm gap (f). (g) Far-field electric field plot ofe. Scale bars, 500 nm. Figure 4: Confined electromagnetic radiation due to anomalous diffraction in anisotropic mesoscale superlattices. ( a ) Simulated 2,000 × 400 nm rod-like superlattice containing dipoles (solid) or a fixed real refractive index value (dashed). Inset depicts the orientation of the superlattices relative to the incident light. ( b ) Effect of changing interparticle gap (volume fraction) on real refractive index of dielectric media ( n =1) with 20 nm Ag spheres. ( c ) Electric field-squared plot of rod-like superlattice with 10 nm surface-to-surface interparticle gap at the extinction maximum (wavelength=645 nm). ( d ) Electric field-squared plot of rod-like superlattice with 60 nm surface-to-surface interparticle gap at the extinction maximum (wavelength=390 nm). ( e ) Absolute electric field plots for 10 nm gap ( e ) and 60 nm gap ( f ). ( g ) Far-field electric field plot of e . Scale bars, 500 nm. Full size image The scattering spectra of the rod-like superlattices are depicted in Fig. 4a (solid lines). Importantly, the maximum peak in the extinction efficiency spectrum is dominated by scattering, such that absorption does not contribute significantly to the main peak, though it does contribute to the extinction near the LSPR of the nanoparticles ( Supplementary Fig. 8 ). Also shown are FDTD (Finite-Difference Time-Domain) simulations of identically shaped structures with real refractive indices chosen to match those from EMT for wavelengths close to the highest peak for a given volume fraction. In Fig. 4b , the real part of the refractive index, n is plotted for the effective media in Fig. 4a . Supplementary Fig. 9 shows the imaginary refractive index, κ , which determines the absorption of light by the superlattice. As expected, κ red shifts with decreasing interparticle separation, accurately describing the red-shift seen when plasmonic nanoparticles come together (in the weak coupling limit, ~1 radius separation) [8] , [53] , [55] . Note that this medium is highly dispersive ( Fig. 4b , red trace) that is, the speed of light changes substantially with wavelength. For a superlattice with Ag 20.2% volume fraction (a 10 nm surface-to-surface gap), the maximum value of n approaches 3 and the minimum is <0.5. Interestingly, the equivalent structure comprising Au nanospheres (rather than Ag) exhibits similar behaviour ( Supplementary Fig. 10 ) where the extinction maximum is shifted far towards the red. However, the additional peaks at shorter wavelength that are seen for Ag are missing for Au, and instead there is a broad peak near the LSPR of the spheres (~520 nm). ADT provides a simple approximation to analyze extinction spectra when the particles are too small for geometric optics [43] . Scattering is approximated well in the limits of anomalous diffraction, that is, l >>λ where l is the path length of light and where the sphere is ‘optically soft’- n near 1. The scattering is driven by phase mismatch between light on the inside and outside of the structures (due to a small refractive index contrast). Maxima in the extinction cross-section occurs when the phase shift is an odd integer times π, that is, Here l is the relevant optical path length, n is the real part of the refractive index and λ is the wavelength. It is important to note that anomalous diffraction expressions have only been developed analytically for a few shapes and that errors of ~20–30% have been observed in applications to water droplets ( n= 1.33) (refs 44 , 45 , 56 ). Using equation (2) with the scattering maximum and mode number as input, an expected refractive index can be calculated. By comparing this with the effective index given by EMT, the error in ADT for these superlattices can be estimated. Table 1 shows the error in the refractive index, which is always < 30% even at the highest volume fraction. This analysis includes higher order ( n =1,3,5) modes and the results are consistent; electric field plots for these are shown in Supplementary Fig. 11 . Note that we exclude the peak in Fig. 4a at ~375 nm because it is not a shape-induced photonic resonance, the electric field profile illustrates that this peak is dominated by the LSPR of the individual nanoparticles. In addition, the error decreases with decreasing volume fraction; this is likely because the effective index becomes less dispersive and closer to 1 near the scattering maximum, diminishing a significant source of error in the ADT approximation. In addition, EMT is less accurate at higher volume fractions because it does not account for electrodynamic interactions. The combination of increased EMT accuracy and the greater validity of the ADT approximation contribute to the smaller error at lower volume fractions, Table 1 , which decreases from (−)20% for the largest volume fraction (10 nm gap) to 6.7% error (20 nm gap), and finally down to 5.3% (30 nm gap). These values are of reasonable accuracy in light of the approximations made in both ADT and EMT. Table 1 Comparison of refractive indices. Full size table In Fig. 4c–f , 2D electric field plots simulated with the CDM are shown for the scattering maxima, depicting both the maximum E 2 value, and the absolute E value, from which phase information can be interpreted. Figure 4c depicts the strongly confined electric field on the interior of the rod at 645 nm, the scattering maximum of the highest volume fraction (20.2%). Notably, this confined electromagnetic mode is absent for the lower volume fraction superlattice ( Fig. 4d , 390 nm). In addition, the scale of the electric field in the superlattice interior is ~20-fold greater when the spheres are separated by one radius (10 nm, Fig. 4c , 20.2% Ag) than when they are separated by 60 nm ( Fig. 4d , 1.0% Ag). Figure 4e depicts the confined nature of the wave; the edge of the superlattices depicts the light ‘bound’ at the interface of the superlattice. Conversely, at the largest 60 nm interparticle gap, shown in Fig. 4f , the wave acts as a leaky fundamental mode, where the electric field is not confined solely to the interior of the superlattice and appears to have an index of 1. Visually it is evident that more wavelengths are able to fit in the superlattice at 1.0% Ag (the lowest volume fraction) compared with the highest volume fraction (20.2%). From this, it is clear that an increased effective index inside of the superlattices will slow down bound waves, maximizing the phase mismatch between the light inside of the structure and the light in vacuum, leading to strong far-field scattering, this is depicted in a far-field projection in Fig. 4g (far-field of Fig. 4e ). Combining Nanoscale and Mesoscale Anisotropy Now consider the combination of nanoscale and mesoscale anisotropy, here focusing on the variation of extinction spectra for ellipsoids with longitudinal excitation (denoted Ell Long ), and for rod-like mesoscale structures with transverse (SL Trans ) or longitudinal (SL Long ) excitation. 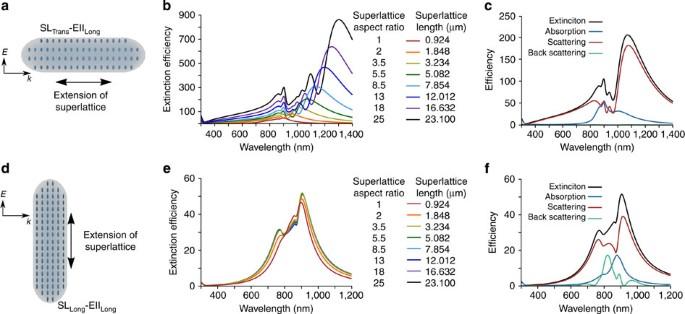Figure 5: Spectral comparison of mesoscale rod-like superlattices composed of longitudinally oriented ellipsoids. (a) Transverse mesoscale superlattice of longitudinally oriented ellipsoids. (b) Spectral change with extension of the mesoscale superlattice shown ina. (c) Spectral decomposition of 5.5AR (b, green trace) into extinction, absorption, scattering and back scattering components. (d) Longitudinal mesoscale superlattice of longitudinally oriented ellipsoids. (e) Spectral change with extension of the mesoscale superlattice shown ind. (f) Spectral decomposition of 5.5 AR (e, green trace) into extinction, absorption, scattering and back scattering. The ellipsoidal inclusions in all simulations are 80 nm long × 10 nm wide at a fixed 80 nm spacing. Figure 5 shows the extinction spectra for a transverse-oriented rod-like superlattice ( Fig. 5a ), SL Trans -Ell Long , with increasing mesoscale aspect ratios (absorption and scattering spectra can be found in Supplementary Fig. 12 ). For simplicity, only the superlattice comprising 8 AR ellipsoids oriented longitudinally are shown. By fixing nanostructure AR, one can isolate the effect of mesoscale shape and orientation on the optical response. In Fig. 5b , as the aspect ratio of the superlattice rod length increases (that is, the rod-like superlattice extends), the major extinction ( λ max ), peak red-shifts. In addition, several periodic peaks indicative of higher order anomalous diffraction modes analogous to those discussed in Fig. 4 emerge blue of the main extinction peak. To determine the nature of the spectral response, it is helpful to decompose the extinction into its absorption, scattering and back-scattering components. Figure 5c depicts the 5.5 AR superlattice optical efficiency spectra ( Fig. 5b , green trace). Again, the main extinction (black trace) resonance peak at ~1,090 nm is dominated by scattering (red trace), analogous to what is seen for spherical nanoparticles in Fig. 4 . In addition, there is a large contribution to the extinction from absorption (blue trace) at 900 nm; this is primarily due to the individual nanoparticle resonances in the interior of the superlattice. ADT and equation (2) explain the periodicity and maxima in the Fig. 5 ; Supplementary Table 2 shows strong agreement between the calculated refractive index using equation (2) and the effective refractive index for 8 AR ellipsoids is shown in Supplementary Fig. 6 . Here, the scattering maximum red shifts due to the extension of the superlattice. This can be explained qualitatively, as the structure extends the light propagates over a larger distance, which increases the phase mismatch between the electric field on the interior and exterior of the structure when it terminates. In addition, the error in Supplementary Table 2 decreases as the extinction maximum shifts towards the red for larger superlattices. This decrease is again due to the real part of the refractive index approaching one at higher wavelengths, where ADT is more accurate. Overall then the behaviour in Fig. 5b can be seen to involve the superposition of a plasmon resonance near 900 nm (see Fig. 2 ) and ADT resonances, which red shift from 900 nm to 1,300 nm as the superlattice AR shifts from 1 to 25. Figure 5: Spectral comparison of mesoscale rod-like superlattices composed of longitudinally oriented ellipsoids. ( a ) Transverse mesoscale superlattice of longitudinally oriented ellipsoids. ( b ) Spectral change with extension of the mesoscale superlattice shown in a . ( c ) Spectral decomposition of 5.5AR ( b , green trace) into extinction, absorption, scattering and back scattering components. ( d ) Longitudinal mesoscale superlattice of longitudinally oriented ellipsoids. ( e ) Spectral change with extension of the mesoscale superlattice shown in d . ( f ) Spectral decomposition of 5.5 AR ( e , green trace) into extinction, absorption, scattering and back scattering. The ellipsoidal inclusions in all simulations are 80 nm long × 10 nm wide at a fixed 80 nm spacing. Full size image In contrast to the transverse mesoscale behaviour in Fig. 5b , the longitudinal rod superlattice orientation ( Fig. 5d ), that is, SL Long -Ell Long , shows that with increasing superlattice aspect ratio, the extinction trend does not change in either resonance location or in peak intensity, Fig. 5e . Again, by looking at the decomposition of the extinction spectrum in Fig. 5f (black trace), we can see that the peak at ~900 nm is dominated by absorption, corresponding to the individual nanoparticle LSPRs, as in Fig. 5c . In addition, a peak further to the red at ~910 nm is primarily scattering driven; this arises from the mesoscale shape and orientation. Because the superlattice only extends longitudinally, and thus the optical depth in the direction of the incident field remains constant as superlattice aspect ratio increases ( Fig. 5d ), we see no change in the scattering resonance location. In addition, there is a significant backscattering component seen between 800 and 900 nm that is not observed in the transverse superlattice orientation (SL Trans ); this behaviour is indicative of an ‘optically metallic’ response discussed in Fig. 3 . A comparison between the electric field profiles for superlattices comprising spheres ( Supplementary Figs 13–16 ) and eight AR ellipsoids ( Supplementary Figs 17,18 ) is also shown. Further elucidation of the spectral differences between a nanorod [57] , [58] and rod-like superlattice is included in Supplementary Note 4 . Superlattices with increasing complexity are described in Fig. 6 . The simplest structure ( Fig. 6a ) is an ~1 micron diameter mesoscale spherical superlattice (SL Sphere ) comprising a simple cubic arrangement of ellipsoidal nanoparticles (separated by one long axis length) of varying aspect ratios. When the ellipsoids have longitudinal orientation (SL Sphere -Ell Long ) to the incident electric field ( Fig. 6a , red), significant red-shifting is seen in the extinction λ max with increasing ellipsoid aspect ratio. By rotating the superlattice 90 degrees, such that the ellipsoids are oriented transverse (SL Sphere -Ell Trans ) to the incident field ( Fig. 6a , blue), the collective superlattice LSPR blue-shifts with increasing aspect ratio. The red-shift is much larger in magnitude than the blue-shift, mimicking the spectral trends seen for individual nanorods [57] . Note that the superlattice sizes here were chosen to minimize shape-induced scattering, such that plasmonic effects dominate the extinction. If the sphere were larger, the extinction would be primarily scattering driven and be readily described by ADT. 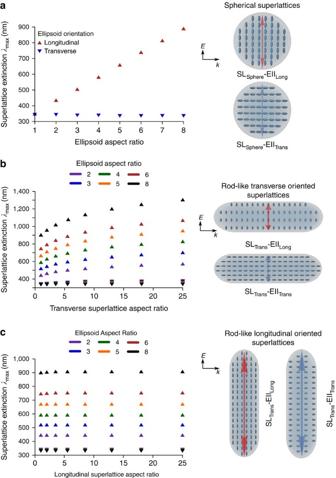Figure 6: Spectral tunability with combined nanoscale and mesoscale anisotropy. (a) Change in the collective optical response (LSPR) of sphere-shaped mesoscale structures comprising ellipsoids with various aspect ratios. (b) Spectral tunability of transverse-oriented superlattices with varying mesostructure aspect ratio (bottom axis) and varying ellipsoidal inclusion aspect ratios (colour). (c) Spectral tunability of longitudinally-oriented superlattices with varying mesostructure aspect ratio (bottom axis) and varying ellipsoidal inclusion aspect ratios (colour). For all plots, longitudinal-oriented ellipsoids are triangles and the transverse-oriented ellipsoids are inverted triangles. Figure 6: Spectral tunability with combined nanoscale and mesoscale anisotropy. ( a ) Change in the collective optical response (LSPR) of sphere-shaped mesoscale structures comprising ellipsoids with various aspect ratios. ( b ) Spectral tunability of transverse-oriented superlattices with varying mesostructure aspect ratio (bottom axis) and varying ellipsoidal inclusion aspect ratios (colour). ( c ) Spectral tunability of longitudinally-oriented superlattices with varying mesostructure aspect ratio (bottom axis) and varying ellipsoidal inclusion aspect ratios (colour). For all plots, longitudinal-oriented ellipsoids are triangles and the transverse-oriented ellipsoids are inverted triangles. Full size image Similar to the structures in Fig. 5 , Fig. 6b,c shows the effect of anisotropy in a mesoscale superlattice structure combined with the spectral tunability provided by the LSPR of high aspect ratio nanoparticle building blocks. With the same varying ellipsoidal inclusions as in Fig. 6a , Fig. 6b considers a rod-like superlattice structure of varying aspect ratio oriented transverse (SL Trans ) to the incident field, and Fig. 6c considers the longitudinal orientation (SL Long ) of the same superlattice. By comparing Fig. 6b,c , the trend with respect to ellipsoid aspect ratio (interior nanoparticles, coloured from purple (two AR) to black (eight AR)) is similar for both rod-like superlattice orientations. Again, a red-shift is seen in the longitudinal ellipsoid orientation (Ell Long ) (triangles) and a blue-shift with the transverse ellipsoid orientation (Ell Trans ) (inverted triangles). From this, we conclude that both superlattice orientation and length determine the path length for optical scattering; further examination of this is included in Supplementary Note 5 . Thus, any desired collective properties identified in the different superlattice orientations can be shifted throughout the visible-NIR. We have demonstrated that, with the incorporation of anisotropy on both the nanoscale and mesoscale, the optical properties of plasmonic nanoparticle superlattices can be rationally designed throughout the UV-visible-NIR. In conjunction with EMT, a new framework of the CDM that incorporates ellipsoids allowed for the fast and efficient simulation of a large variety of plasmonic superstructures. It is shown that control of nanoparticle structure can produce a superlattice crystal that exhibits both birefringence (polarization dependence) and is dichromatic (properties dependent on crystal orientation), independent of the superlattice mesostructure. However, the mesoscale structure can also profoundly affect the optical properties, with transverse orientation leading to strong directionally confined electromagnetic fields, and longitudinal orientation featuring ENZ and ‘optically metallic’ behaviour, as can be described by EMT. The mesoscale effects observed in superlattices can be interpreted using the simple combination of EMT with ADT, which is confirmed with numerical coupled dipole and FDTD simulations. This proof-of-concept that the collective optical properties of a superstructure can be determined by combining nanoscale nearest neighbour assembly and mesoscale shape control of plasmonic nanoparticle superlattices will help guide future assembly techniques and architectures. The ability to manipulate and guide light at and below the diffraction limit is relevant to a variety of applications centered around optical electronics [59] , electromagnetic field enhancement [60] , [61] , light concentration [60] , [62] and visible light metamaterials [63] , [64] , [65] . We envision that these results will aid in merging the vast array of nanoscale synthesis and assembly techniques with the increasingly well-understood and exciting properties of metamaterials. Maxwell-Garnett Effective Medium Theory To develop an effective medium approximation, we consider a low volume fraction of inclusions where electrodynamic interactions between the nanoparticles are minimal. Assuming that the ellipsoid axes are aligned, the collective material properties can be described by an effective dielectric function ε eff : where ε is the dielectric function of the material and f is the volume fraction of the metal inclusions, given by: where N is the number of nanoparticle inclusions per unit cell, V nanoparticle is the metal volume of each nanoparticle and V unit cell is the total volume of interest, in this case a single unit cell. Coupled Dipole Method Various methods for the simulation of noble metal nanoparticles exist including finite element methods (FEM), the discrete dipole approximation (DDA) [10] , [66] and finite difference time-domain (FDTD), among others. For the treatment of superlattice structures, we have demonstrated that the CDM [53] , [55] (CDM, closely related to DDA for our implementation) correlates well with experimental results for DNA-nanoparticle materials [8] , [53] , [55] , [67] . This method provides an extremely fast method for the simulation of aggregates of metal nanospheres with both arbitrary nearest neighbour symmetries and arbitrary superstructure shape. Within the CDM, a superlattice material is represented as a lattice of dipoles, where the induced dipole in each particle is treated in the quasistatic approximation, yet the interactions between dipoles are fully retarded. Using the open-source DDSCAT [68] , [69] code, the dipole-dipole interactions are evaluated using Fast Fourier Transforms. In brief, in the CDM, the polarization P i of the i th dipole is given by where E loc ( r i ) is the sum of the incident plane wave and the electric field generated by all the other dipoles at a given point, r i . For a sphere, the polarizability of a single dipole α i is given by the quasistatic expression where ε is the complex, frequency dependent dielectric function of the metal, ε b is the dielectric constant of the background media and a is the volume of a sphere ( a= 4/3 πr 3 ). In principle, this same approach can be used to simulate other shapes such as ellipsoids, which we use to approximate a rod. However, the quasistatic approximation is only appropriate for rods with long axes up to a 100 nm and short axes up to 20 nm. Above this size, the retarded fields inside the structure need to be accounted for [70] . The polarizability of an ellipsoid is easily described in the quasistatic limit as: where L is the geometrical factor, whose inputs are the long and short radii of the ellipsoid and V is the volume of the ellipsoid, 4/3 πab 2 , where a and b are the long and short axes lengths, respectively. Note that for a sphere, L=1/3 and this expression reduces to the quasistatic result for sphere (equation (6)). The geometrical factor, L, for the longitudinal mode of an ellipsoid is described by where e is the eccentricity of the ellipsoid, where a (long axis) and b (short axis) are input, Because the sum of the total geometrical factor must equal 1 and that the two transverse modes are degenerate, the transverse geometrical factor can be determined from How to cite this article : Ross, M. B. et al. Using nanoscale and mesoscale anisotropy to engineer the optical response of three-dimensional plasmonic metamaterials. Nat. Commun. 5:4090 doi: 10.1038/ncomms5090 (2014).